A water-soluble nucleolin aptamer-paclitaxel conjugate for tumor-specific targeting in ovarian cancer Paclitaxel (PTX) is among the most commonly used first-line drugs for cancer chemotherapy. However, its poor water solubility and indiscriminate distribution in normal tissues remain clinical challenges. Here we design and synthesize a highly water-soluble nucleolin aptamer-paclitaxel conjugate (NucA-PTX) that selectively delivers PTX to the tumor site. By connecting a tumor-targeting nucleolin aptamer (NucA) to the active hydroxyl group at 2′ position of PTX via a cathepsin B sensitive dipeptide bond, NucA-PTX remains stable and inactive in the circulation. NucA facilitates the uptake of the conjugated PTX specifically in tumor cells. Once inside cells, the dipeptide bond linker of NucA-PTX is cleaved by cathepsin B and then the conjugated PTX is released for action. The NucA modification assists the selective accumulation of the conjugated PTX in ovarian tumor tissue rather than normal tissues, and subsequently resulting in notably improved antitumor activity and reduced toxicity. Paclitaxel (PTX) is one of the most commonly used first-line drug for treating a variety of cancers in clinical chemotherapy [1] , [2] . However, its poor water solubility restricts its direct clinical applications [3] . More importantly, PTX does not explicitly discriminate between cancer cells and normal cells and frequently leads to serious undesirable side effects [4] , [5] . Attaching to tumor recognition elements has been proven beneficial for selective delivery of anti-cancer compounds to tumor cells; however, few tumor-targeting elements was proved to be successful. Although some antibody-drug conjugates (ADCs) have been approved for clinical treatment, there are still challenges when utilizing antibodies for drug delivery, especially the risk of immunogenicity and the raising incidents of resistance [6] , [7] , [8] , [9] . In addition, difficulties in synthesis and chemical modification, and rigorous storage requirement are also the major concerns [8] . Therefore, it is highly desirable to develop paclitaxel derivatives with tumor-targeting property. Nucleic acid aptamers are small single-stranded DNA or RNA oligonucleotide segments, which bind to their targets, such as proteins with high affinity and specificity by unique three-dimensional (3D) structure [10] , [11] , [12] , [13] . Aptamers have been widely used as tumor recognition elements [13] . In contrast to antibodies, aptamers have limited immunogenicity and are unlikely to develop resistance [11] , [14] , [15] . Besides, rapid targeted cell penetration and excellent stability of aptamers are also desired advantages [16] , [17] . As one of the most successful tumor-targeted aptamers [18] , [19] , a nucleolin aptamer (AS1411, NucA) in phase II trial (NCT00740441) for treating metastatic renal cell carcinoma has been confirmed with excellent tumor-targeting property and exceptional safety [20] . NucA interacts with nucleolin protein, which normally locates in the nucleus; however, also found expressing on the surface of cancer cells [19] . Hence, NucA could be a promising tumor-targeting element for developing paclitaxel derivatives. Cathepsin B is an intracellular lysosomal protease and its general substrates include valine-citrulline and phenylalanine-arginine [21] . Cathepsin B mainly locates in lysosomes with a favorable pH from 4.5 to 5.0 [22] , and plays an important role in invasion and metastasis in tumor cells [23] , [24] . The trace amount of cathepsin B in blood circulation normally stays inactive due to unfavorable pH conditions and the existence of protease inhibitors. Therefore, via a cathepsin B-labile valine-citrulline dipeptide linker, the tumor-targeting NucA can be connected to PTX at the C-2′ position as a nucleolin aptamer-paclitaxel conjugate (NucA-PTX). The intact NucA-PTX is supposed to have no or low activity as the substitution of 2′-hydroxyl group on PTX with other groups resulted in the loss of antitumor activity for the PTX derivative [25] . The conjugate is postulated to remain stable in blood circulation, whereas once delivered to tumor cells via NucA recognition to the cell surface nucleolin and taken up by endocytosis, the linker can be cleaved by lysosomal proteases in tumors, resulting in PTX release for action. To ensure the complete release of PTX, p -aminobenzylcarbonyl (PABC) can be incorporated between PTX and the dipeptide linker, which facilitates the conjugate being hydrolyzed and releasing PTX through spontaneous 1,6-elimination reaction. On the other side, succinic acid can be introduced to reduce the steric hindrance between NucA and the dipeptide linker, which facilitates not only the enzymolysis of the linker by cathepsin B, and also the binding of NucA to nucleolin. In this study, we synthesize the designed NucA-PTX which shows both good water solubility and tumor-targeting property. By utilizing a Fluorescein amidate (FAM) and Rhodamine B (Rh) dual-labeled conjugate (FAM-NucA-PTX-Rd) with fluorescence resonance energy transfer (FRET) existing between two fluorophores, the stability of NucA-PTX in human serum and the release of the conjugated PTX in tumor are verified. Moreover, the PTX conjugation does not considerably affect the binding affinity between NucA and its target protein nucleolin, which is supported by both molecular dynamic simulation and isothermal titration calorimetry (ITC). The NucA modification is shown to facilitate the uptake of the conjugated PTX in ovarian cancer cells mainly by macropinocytosis in a nucleolin expression-dependent manner, leading to higher cytotoxicity of the conjugated PTX to ovarian cancer cells compared to normal cells. The in vivo data collected from a human xenograft model of ovarian cancer demonstrated that the NucA modification facilitates the selective accumulation of the conjugated PTX in ovarian tumor tissue, and subsequently resulting in notably improved antitumor activity and reduced toxicity. Synthesis of aptamer-paclitaxel conjugates Synthesis of NucA-PTX ( 7a , Fig. 1 ) commenced with 1 and PABOH in the presence of EEDQ to provide 2 . Then 3 was produced by treating 2 with PNP chloroformate in the presence of pyridine. Transesterification of p -nitrophenoxy on 3 with PTX under the catalytic condition of DMAP afforded 4 . The Fmoc protecting group in 4 was quickly removed by piperidine in DMF, giving rise to 5 . Without further purification, the amino group in 5 was reacted with succinic anhydride in the presence of DIPEA, providing 6 with a free carboxyl group. 6 was then conjugated with NucA in the presence of Sulfo-NHS and EDCI to afford NucA-PTX ( 7a ). CRO-PTX ( 7b ) was prepared as described above by using a control aptamer CRO (C-rich oligonucleotide) for conjugation at the last step (Fig. 1 ). The structures of key intermediates were confirmed by 1 H-NMR, 13 C-NMR, 2D [ 1 H, 1 H] COSY spectroscopy and high-resolution mass spectrometry (Supplementary Figs. 1 − 4 ). NucA-PTX was characterized by HPLC, mass spectrometry and 1 H-NMR, 2D [ 1 H, 1 H] COSY, 2D [ 1 H, 1 H] NOESY spectroscopy (Supplementary Figs. 5, 6 ). The structure of CRO-PTX was confirmed by HPLC and mass spectrometry (Supplementary Fig. 7 ). To synthesize PTX-Rh (Supplementary Fig. 17 ), the 2′-hydroxyl group on PTX was protected by TBS in the presence of TBSCl and imidazole to afford 8 in good yield. Treated with Rhodamine B, 8 was converted into 9 upon formation of ester group in the presence of EDCI and DMAP. The free 2′-hydroxyl group of 10 was obtained after deprotection of TBS group using hydrogen fluoride-pyridine. Compounds 11 , 12 , 13 , FAM-NucA-PTX-Rh ( 14a ), NucA-PTX-Rh ( 14b ), and CRO-PTX-Rh ( 14c ) were prepared with the same method as described above. The structures of key intermediates were confirmed by 1 H-NMR, 13 C-NMR spectroscopy and high-resolution mass spectrometry, and the conjugates were confirmed by HPLC and mass spectrometry (Supplementary Figs. 8 − 15 ). The water solubility of NucA-PTX was significant improved compared to that of free PTX (Supplementary Fig. 18 ). Fig. 1 Synthesis of aptamer-paclitaxel conjugates. Note for reagents and conditions: (i) PABOH, EEDQ, CH 2 Cl 2 /CH 3 OH; (ii) PNP chloroformate, pyridine, THF; (iii) PTX, DMAP, CH 2 Cl 2 ; (iv) piperidine, DMF; (v) succinic anhydride, DIPEA, THF; (vi) Sulfo-NHS, EDCI, aptamer, dd-H 2 O, DMF, 0.5 M Na 2 CO 3 /NaHCO 3 . Fmoc = 9-Fluorenylmethoxycarbonyl, PABOH = 4-Aminophenylmethanol, EEDQ = N -ethoxycarbonyl-2-ethoxy-1,2-dihydroquinoline, PNP = p -Nitrophenyl, DMAP = 4-Dimethylaminopyridine, Bz = Benzoyl, Ac = Acetyl, DMF = Dimethylformamide, DIPEA = N , N′ -Diisopropylethylamine, THF = Tetrahydrofuran, Sulfo-NHS = N -hydroxysulfosuccinimide sodium salt, EDCI = 1-Ethyl-3-(3-dimethyllaminopropyl)carbodiimide hydrochloride, NucA = Nucleolin aptamer, CRO = Cytosine-rich oligonucleotide Full size image The stability of NucA-PTX and the release of paclitaxel To verify the stability of NucA-PTX in circulation and the intracellular release of PTX, a dual fluorophore-labeled conjugate—FAM-NucA-PTX-Rh was designed according to the fluorescence resonance energy transfer (FRET) principle (Fig. 2a ). Fluorescein amidate (FAM) was linked to the 5′ end of NucA as the donor and rhodamine B (Rh) was linked to the 7-hydroxyl group of PTX as the acceptor. When the dipeptide linker stays intact, the fluorescence of both fluorophores in FAM-NucA-PTX-Rh remained stable. Whereas when the linker is hydrolyzed in the presence of the specific protease—cathepsin B, FRET between FAM and rhodamine B is interrupted, appeared as the decrease of Rh intensity and the increase of FAM intensity. With an excitation wavelength at 470 nm, FRET was noted in the fluorescence emission spectrum of FAM-NucA-PTX-Rh compared to the individual spectra of FAM-NucA and PTX-Rh (Fig. 2b ). Whereas, in the presence of cathepsin B, increased emission at 520 nm and decreased emission at 590 nm upon time were observed in the spectra of FAM-NucA-PTX-Rh (Fig. 2c ). Accordingly, the concentration of intact FAM-NucA-PTX-Rh could be presented by the fluorescence intensity ratio at 590 nm and 520 nm (RFI λ 590 / λ 520 ), while the concentration of free PTX-Rh could be inversely reflected by the fluorescence intensity at 590 nm (FI λ 590 ). When FAM-NucA-PTX-Rh was incubated in human serum at 37 °C for 48 h, both RFI λ 590 / λ 520 and FI λ 590 remained the same upon time (Fig. 2d ), suggesting FAM-NucA-PTX-Rh existed as the intact form. In contrast, in a buffered solution of cathepsin B (pH 5.0), both RFI λ 590 / λ 520 and FI λ 590 decreased upon time, while those in buffer without cathepsin B remained unchanged (Fig. 2d ), implying the successful cleavage of the linker and the release of free PTX-Rh. The stability and dissociation of NucA-PTX were confirmed by HPLC analysis with consistent results (Supplementary Fig. 19 ). To further probe the intracellular release of PTX-Rh from FAM-NucA-PTX-Rh in ovarian cancer cells, SKOV3 cells were treated with FAM-NucA-PTX-Rh and the fluorescence of FAM and Rh of the cells at 1, 3, and 6 h was analyzed by flow cytometry. In consistence of the results obtained extracellularly (Fig. 2d ), the relative fluorescence intensity RFI (Rh/FAM) kept decreasing upon time (Fig. 2e ), implying the successful intracellular release of PTX-Rh from NucA-PTX. Fig. 2 The cathepsin B-dependent release of PTX in FAM-NucA-PTX-Rh. a Schematic diagram of the utilization of FRET in FAM-NucA-PTX-Rh for tracking the rupture of the cathepsin B-labile linker. b Fluorescence emission spectra of FAM-NucA-PTX-Rh, FAM-NucA and PTX-Rh ( λ ex = 470 nm). All compounds were at a concentration of 2 μM. c Fluorescence emission spectra of FAM-NucA-PTX-Rh ( λ ex = 470 nm) in the presence of cathepsin B upon time. FAM-NucA-PTX-Rh and cathepsin B were at a concentration of 2 μM and 0.5 unit mL −1 , respectively. d The fluorescence analysis of FAM-NucA-PTX-Rh in human serum and buffer (pH 5.0, containing DTT) without or with cathepsin B upon time. The relative fluorescence intensity of rhodamine to FAM (RFI λ 590 / λ 520 ) indicates the concentration of FAM-NucA-PTX-Rh, and the fluorescence intensity of rhodamine (FI λ 590 ) indicates the concentration of the conjugated PTX-Rh. FAM-NucA-PTX-Rh and cathepsin B were at a concentration of 2 μM and 0.5 unit mL −1 , respectively. Error bars indicate mean ± standard deviation. n = 3. e The intracellular release of PTX-Rh from FAM-NucA-PTX-Rh in SKOV3 cells monitored by flow cytometry. The relative median fluorescence intensity of rhodamine to FAM (RFI Rh/FAM) in SKOV3 cells was examined 1, 3, and 6 h after incubation with 200 nM FAM-NucA-PTX-Rh. Error bars indicate mean ± standard deviation. n = 3, * P < 0.05 Full size image The effect of PTX on NucA and nucleolin interaction Nucleolin binding is essential for achieving the tumor-targeting property of NucA-PTX. To investigate whether the conjugated PTX affects the interaction between NucA and its target protein nucleolin, their binding affinity before and after PTX conjugation was studied by both molecular dynamic simulation and isothermal titration calorimetry (ITC). Nucleolin of eukaryotic cell comprises several domains, including an acidic N-terminal domain, four RNA binding domains (RBD) and a C-terminal RGG-rich “tail” (Supplementary Fig. 20a ). In the simulated model, we found that both NucA and NucA-PTX conjugate interacted with RGG-rich domain of the C-terminal of nucleolin, which was consistent with previously reported [26] . Structurally, the conjugated PTX segment laid at the end of the chain in the simulated model (Supplementary Fig. 20b ). Quantitatively, no considerable difference was observed in the calculated binding free energy between NucA and NucA-PTX conjugate when docking to nucleolin. Moreover, the binding of NucA or NucA-PTX with Nucleolin was examined using isothermal titration calorimetry. By titrating NucA or NucA-PTX into the nucleolin protein solution with a 10:1 ratio of concentration, results demonstrated that the PTX conjugation did not significantly affect the interaction between NucA and nucleolin ( Fig. 3a ) , with the K d value 151 ± 24 nM before conjugation and 267 ± 43 nM after conjugation, respectively. Fig. 3 The effect of NucA modification on the uptake of the conjugated PTX-Rh. a The interaction of nucleolin with NucA and NucA-PTX, respectively, detected by isothermal titration calorimetry (ITC). NucA or NucA-PTX was injected into nucleolin at a 10:1 ratio in 19 portions (each portion 2 μL) at 25 °C. b The time-dependent cellular uptake of the conjugated PTX-Rh in SKOV3 cells examined by flow cytometry. SKOV3 cells were incubated with either NucA-PTX-Rh or CRO-PTX-Rh at a concentration of 500 nM for 1 to 6 h. Error bars indicate mean ± standard deviation. n = 5, * P < 0.05. c The concentration-dependent cellular uptake of the conjugated PTX-Rh in SKOV3 cells examined by flow cytometry. SKOV3 cells were incubated with either NucA-PTX-Rh or CRO-PTX-Rh at a range of concentrations for 2 h. Error bars indicate mean ± standard deviation. n = 5, * P < 0.05. d The nucleolin expression on cell surface, and the uptake of NucA-PTX-Rh or CRO-PTX-Rh in SKOV3, OVCAR3 and L02 evaluated by flow cytometry. The cells were treated with NucA-PTX-Rh or CRO-PTX-Rh at a concentration of 100 nM for 2 h. The nucleolin expression was detected using Alexa488-labeled anti-nucleolin antibody shown in the FITC channel, and the rhodamine level of the conjugates was shown in the PE channel. e The cellular uptake of NucA-PTX-Rh in SKOV3 pre-incubated with either NucA (NucA Pre) or CRO (CRO Pre) analyzed by flow cytometry. The cells were pretreated with 250 nM NucA or CRO for 2 h before incubated with 100 nM NucA-PTX-Rh for 2 h. The rhodamine level of NucA-PTX-Rh was shown in the PE channel Full size image The effect of NucA modification on cellular uptake The uptake of NucA-PTX-Rh or CRO-PTX-Rh in SKOV3 cells was examined by detecting the rhodamine fluorescence intensities in SKOV3 cells using flow cytometry. The uptake of NucA-PTX-Rh in SKOV3 cells was shown to increase upon time and concentration, which was significantly higher than that of its counterpart CRO-PTX-Rh (Fig. 3b, c ). To examine whether the uptake of the conjugated PTX-Rh was nucleolin-dependent, the uptake of NucA-PTX-Rh in three cell lines: two human ovarian cancer cell lines—SKOV3 and OVCAR3, and one human normal liver cell line—L02 were examined in this study. Different expression levels of nucleolin on the cell surface were observed for the three cell lines, with L02 the lowest and SKOV3 the highest ( Fig. 3d ). The uptake of NucA-PTX-Rh in the three cell lines was found increasing along with the nucleolin expression. The highest uptake of NucA-PTX-Rh was observed in SKOV3 cells with the top nucleolin expression, and the lowest uptake in L02 cells with the least nucleolin expression (Fig. 3d ). In contrast, the uptake of CRO-PTX-Rh did not vary significantly among the three cell lines ( Fig. 3d ), implying the specificity of NucA targeting. When the nucleolin on SKOV3 cells were partially blocked by preincubation with NucA, the uptake of NucA-PTX showed a significant decrease (Fig. 3e ). While the preincubation with CRO aptamer resulted in a less blocking effect and consequently a smaller decrease of NucA-PTX-Rh uptake (Fig. 3e ), further suggesting the uptake of NucA-PTX-Rh in cells was correlated with available nucleolin on the cell surface. It is noteworthy that there was considerable amount of uptake for CRO-PTX-Rh in SKOV3 cells; however, its indiscriminate uptake in other cell lines with different nucleolin surface expressions suggested that the uptake of CRO-PTX-Rh was non-specific and nucleolin-independent (Fig. 3b–d ). The effect of NucA modification on cellular internalization To explore whether the conjugated PTX was taken up by SKOV3 cells through endocytosis resulted from the NucA modification, SKOV3 cells was incubated with NucA-PTX-Rh or CRO-PTX-Rh in the presence of Alexa Fluor 488-labeled endocytic markers and analyzed by confocal microscopy. The quantification of the co-localization of the conjugated PTX and endocytic markers was carried out using Pearson’s correlation coefficient analysis by ImageJ. A remarkable co-localization of NucA-PTX-Rh with Dextran (a marker for macropinocytosis) in SKOV3 cells was observed (Fig. 4a ), with Pearson’s correlation coefficient ~0.8 (Fig. 4b ). In contrast, a significant lower co-localization of NucA-PTX-Rh with transferrin (a marker for clathrin-mediated endocytosis) or choleratoxin (a marker for caveolae-mediated endocytosis) were detected (Fig. 4a, b ), indicating that NucA-PTX-Rh was mainly taken up by SKOV3 cells via macropinocytosis. This was also confirmed by the reduced uptake of NucA-PTX-Rh when cells were pretreated with EIPA (an inhibitor of macropinocytosis) at various concentrations (Fig. 4c ), while the uptake was not substantially affected by the inhibition of the other two pathways (Fig. 4d, e ). The distribution of CRO-PTX-Rh in SKOV3 cells was more dispersed compared to that of NucA-PTX-Rh, and no significant co-localization of CRO-PTX-Rh with any of the three markers was observed (Supplementary Fig. 22a, b ). The inhibition of three endocytic pathways did not dramatically affect the uptake of CRO-PTX-Rh (Supplementary Fig. 22c ), implying the non-specific uptake of CRO-PTX-Rh in SKOV3 cells. The cellular trafficking of NucA-PTX-Rh in SKOV3 cells after macropinocytosis was then presented by the predominant co-localization of NucA-PTX-Rh with lysotrackers in contrast to its CRO counterpart (Fig. 4f, g ). The lysosome transportation for NucA-PTX-Rh could facilitate the rupture of the cathepsin B-labile linker in the conjugate in the presence of lysosomal cathepsin B and efficiently release PTX. In addition, the co-localization of NucA-PTX-Rh with endocytic markers in L02 cells were also investigated. The lack of co-localization with any of the endocytic markers and the unaltered uptake by all endocytic pathway inhibitors were also noted (Supplementary Fig. 23 ). Hence, endocytosis of NucA-PTX-Rh in normal cells was unlikely involved and the uptake could be much less efficient than that in cancerous cells. Fig. 4 The effect of NucA modification on cellular internalization and trafficking. a Representative images showing the co-localization of the conjugated PTX-Rh (red) in NucA-PTX-Rh with Alexa Fluor 488-labled endocytic markers (transferrin, choleratoxin and dextran; green) by confocal microscopy. The nuclei were counterstained with Hoechst 33,342 (blue). Scale bar, 10 μm. b Pearson’s correlation coefficient analysis of the co-localization between NucA-PTX-Rh and endocytosis markers in SKOV3 cells by Image J Coloc2. Error bars indicate mean ± standard deviation. n = 5 per group. Each replicate is from one biological experiment, quantified with 10 independent fields of view. * P < 0.05; NS: not significant difference. c - e The chemical inhibition of cellular uptake for the conjugated PTX-Rh in CRO-PTX-Rh in SKOV3 cells. The relative fluorescence of rhodamine was quantified after the treatment with inhibitors of three endocytic pathways by flow cytometry: EIPA (macropinocytosis, c ), Filipin (caveolae pathway, d ), and Chlorpromazine (clathrin pathway, e ). Error bars indicate mean ± standard deviation. n = 3. * P < 0.05; NS: not significant difference. f Representative images showing the co-localization of the conjugated PTX-Rh (red) with a lysosomal marker (LysoTracker Green DND-26; green) by confocal microscopy. The nuclei were counterstained with Hoechst 33,342 (blue). Scale bar, 10 μm. g Pearson’s correlation coefficient analysis of the co-localization between the conjugates and lysotracker in SKOV3 cells by Image J Coloc2. The data were presented as the means ± standard deviation. n = 5 per group. Each replicate is from one biological experiment, quantified with 10 independent fields of view. * P < 0.05 Full size image The effect of NucA modification on the cytotoxicity To examine whether the NucA modification affects the antitumor activity of the conjugated PTX in ovarian cancer cells, the 24 h and 72 h cytotoxicity of NucA-PTX, CRO-PTX, PTX, NucA, and CRO on two human ovarian cancer cell lines—SKOV3 and OVCAR3, and a normal liver cell line—L02, was examined using Cell Counting Kit-8 (CCK8). 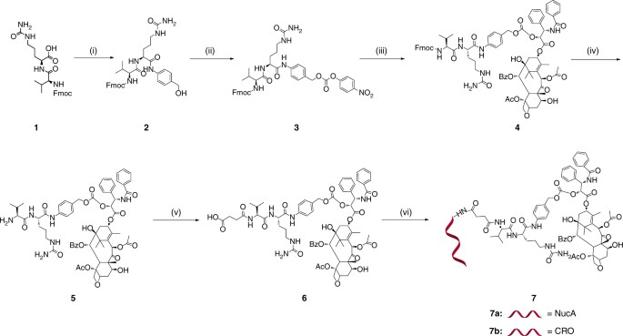Fig. 1 Synthesis of aptamer-paclitaxel conjugates. Note for reagents and conditions: (i) PABOH, EEDQ, CH2Cl2/CH3OH; (ii) PNP chloroformate, pyridine, THF; (iii) PTX, DMAP, CH2Cl2; (iv) piperidine, DMF; (v) succinic anhydride, DIPEA, THF; (vi) Sulfo-NHS, EDCI, aptamer, dd-H2O, DMF, 0.5 M Na2CO3/NaHCO3. Fmoc = 9-Fluorenylmethoxycarbonyl, PABOH = 4-Aminophenylmethanol, EEDQ =N-ethoxycarbonyl-2-ethoxy-1,2-dihydroquinoline, PNP =p-Nitrophenyl, DMAP = 4-Dimethylaminopyridine, Bz = Benzoyl, Ac = Acetyl, DMF = Dimethylformamide, DIPEA =N,N′-Diisopropylethylamine, THF = Tetrahydrofuran, Sulfo-NHS =N-hydroxysulfosuccinimide sodium salt, EDCI = 1-Ethyl-3-(3-dimethyllaminopropyl)carbodiimide hydrochloride, NucA = Nucleolin aptamer, CRO = Cytosine-rich oligonucleotide The IC 50 values at 72 h is shown in Supplementary Table 1 . For two ovarian cancer cell lines, NucA-PTX exhibited comparable cytotoxicity as PTX but higher cytotoxicity than CRO-PTX (Fig. 5a , Supplementary Fig. 24 , Supplementary Table 1 ). When it comes to the normal liver cell line L02, though NucA-PTX had a slightly inhibitory effect on cell proliferation, it was still significantly less cytotoxic compared to CRO-PTX or PTX ( Fig. 5a , Supplementary Fig. 24 , Supplementary Table 1 ) . The cytotoxicity of NucA-PTX to L02 was less than that to cancer cell lines. NucA and CRO exhibited no considerable cytotoxicity in all cell lines within the concentration range examined (Fig. 5a , Supplementary Fig. 24 ). Furthermore, the effect of NucA-PTX on cell cycle was also investigated. NucA-PTX increased the fraction of cells in G2/M phase in the cell cycle of SKOV3 and OVCAR3 as PTX did after 48 h treatment; however, for CRO-PTX the majority of cells were still in G0/G1 phase (Fig. 5b ), which is consistent with the cytotoxicity results. Fig. 5 The effect of NucA modification on the cytotoxicity of the conjugated PTX. a The cell viabilities of SKOV3, OVCAR3, and L02 after 24 h treatment of NucA, CRO, PTX, CRO-PTX, or NucA-PTX evaluated by CCK8 assay. The concentration range of each compound was from 15.6 to 500 nM. The data were presented as the means ± standard deviation. n = 3. b The cell cycle distribution of SKOV3 and OVCAR3 cells after 48 h treatment of CRO-PTX, NucA-PTX, or PTX analyzed by flow cytometry Full size image The effect of NucA modification on in vivo distribution To examine the tumor-targeting property of the NucA conjugated PTX-Rh, the tissue distribution of PTX-Rh was evaluated in a xenografted mice model of human ovarian cancer by biophotonic imaging. It was shown that the Rh fluorescence intensities in ovarian tumor tissues collected from the NucA-PTX-Rh treated mice were significantly higher than those from the CRO-PTX-Rh treated mice at 2 h and 4 h after intravenous injection of NucA-PTX-Rh and CRO-PTX-Rh, respectively (Fig. 6a ). Moreover, the Rh fluorescence intensities in livers and kidneys from the NucA-PTX-Rh treated mice were remarkably lower when compared to those from the CRO-PTX-Rh treated mice at 4 h after injection (Fig. 6a ). Interestingly, the fluorescence signal was hardly detected in hearts, spleens and lungs in both groups (Fig. 6a ). The percentage of injected dose of NucA-PTX-Rh and CRO-PTX-Rh in tumor and other major viscera at 2 h and 4 h were also analyzed to quantitatively examine the effect of NucA on the distribution of the conjugated PTX-Rh. In consistency, the accumulation of NucA-PTX-Rh in tumor was significantly higher than that CRO-PTX-Rh at both time points, while the clearance of NucA-PTX-Rh in liver and kidney at 4 h was considerably faster (Fig. 6b ). The serum half-life of NucA-PTX-Rh was evaluated to be ~2.17 h (Supplementary Fig. 25 ). To further confirm whether NucA could selectively deliver the conjugated PTX-Rh into tumor cells on which nucleolin was highly expressed, we examined the co-localization of PTX-Rh with the nucleolin-expressing cells in the tumor cryosections from the xenografted mice injected with NucA-PTX-Rh or CRO-PTX-Rh by immunofluorescent analysis with confocal imaging. Although there were numerous instances of nucleolin-expressing cells in the tumor cryosections of both groups, more co-localization of Rh fluorescent signal with nucleolin-expressing cells were found in the NucA-PTX-Rh-treated mice as compared to the CRO-PTX-Rh treated mice at 4 h after injection (Fig. 6c, d ). In addition, there were lower percentages of nephrocytes and hepatocytes with Rh fluorescent signal (Rh+ cells) per microscopic view in the NucA-PTX-Rh-treated mice as compared to the CRO-PTX-Rh treated mice at 4 h after injection (Fig. 6e, f ). Furthermore, we wonder whether the linker of NucA-PTX-Rh remained intact when the conjugate reached the tumor site, which is crucial for the tumor-specific accumulation of the conjugated PTX. After a single dose of NucA-PTX-Rh and FAM-NucA-PTX-Rh, the fluorescence of rhoamine in NucA-PTX-Rh treated mouse tumors (representing the concentration of PTX-Rh in the conjugate) and the fluorescence of rhodamine and FAM in FAM-NucA-PTX-Rh treated mouse tumors (FAM/Rh representing the intact conjugate illustrated in Fig. 2 ) were analyzed. The PTX-Rh gradually accumulated in tumor tissue in the first 2 h after injection, and started being cleared from the tissue after 2 h (Supplementary Fig. 26a ). Interestingly, the relative fluorescence intensity (RFI) Rh/FAM exhibited a plateau at the beginning, and then gradually decreased after 2 h (Supplementary Fig. 26b ). The initial plateau of RFI Rh/FAM could be explained by the continuous accumulation of intact conjugate at the tumor site. The subsequent reduction of RFI Rh/FAM could possibly because when there was no accumulation of new intact conjugate after 2 h, the release of PTX-Rh from the conjugate in the tumor tissue could be observed. Fig. 6 The effect of NucA modification on the distribution of the conjugated PTX-Rh. a The distribution of the conjugated PTX-Rh in tumor and major viscera (heart, liver, spleen, lung, and kidney) at organ level 2 h and 4 h after intravenous injection of NucA-PTX-Rh or CRO-PTX-Rh visualized by biophotonic imaging. b Percentage of injected dose in tumor and major viscera 2 h and 4 h after intravenous injection of NucA-PTX-Rh or CRO-PTX-Rh evaluated by measuring the fluorescent intensity of rhodamine. The data were presented as the means ± standard deviation. n = 6, NS: not significant, * P < 0.05. c The representative fluorescent micrographs of the distribution of the conjugated PTX-Rh in tumor at tissue level 4 h after intravenous injection of NucA-PTX-Rh or CRO-PTX-Rh examined by confocal microscopy. NucA-PTX-Rh and CRO-PTX-Rh were indicated by rhodamine (red). Immunofluorescence staining was performed by Alexa488-labeled anti-nucleolin antibody (green). Merged images with DAPI staining show co-localization of the conjugates with nucleolin positive cells. H&E staining images were from the same cryosections. Scale bars, 80 μm. d The Pearson’s coefficient analysis for the distribution of the conjugated PTX-Rh (red) with nucleolin-expressing tumor cells (green). e Representative fluorescent micrographs of the distribution of the conjugated PTX-Rh in kidney and liver at tissue level 4 h after intravenous injection of NucA-PTX-Rh or CRO-PTX-Rh examined by confocal microscopy. NucA-PTX-Rh and CRO-PTX-Rh were indicated by rhodamine (red). Merged images with DAPI staining show rhodamine positive cells. H&E staining images were from the same cryosections. Scale bars, 80 μm. f The percentage of rhodamine positive cells per microscopic view. Note: CRO-PTX-Rh, the xenografted mice treated with CRO-PTX-Rh. NucA-PTX-Rh, the xenografted mice treated with NucA-PTX-Rh. The data were presented as the means ± standard deviation. n = 4, * P < 0.05 vs. CRO-PTX-Rh group Full size image The effect of NucA modification on in vivo efficacy The in vivo antitumor effect of NucA-PTX was evaluated in a xenografted mice model of human ovarian cancer. Compared with PBS-treated group (control group) and CRO-treated group (aptamer control group), the others groups exhibited significantly lower tumor volumes, wherein the NucA-PTX treated group showed a better inhibitory effect against tumor growth that PTX-treated group or nucleolin aptamer-treated group (Fig. 7a ). Especially, the average tumor volume of the NucA-PTX treated group was significantly smaller than that treated with PTX and other groups ( P < 0.05) on day 28 (Fig. 7b ). Then, Ki-67 antigen staining, a commonly used cell proliferation marker, together with H&E staining, were performed to further investigate the tumor suppression efficiency of NucA-PTX. For Ki-67 staining, we found numerous instances of Ki-67-positive cells in tumor tissue from PBS-treated and aptamer-treated xenografted mice, indicating active cell proliferation. In contrast, the NucA-PTX treated group showed a lower Ki-67-positive cells than PTX treated groups and the other control groups (Fig. 7c ), suggesting a higher inhibition effect on tumor growth. For H&E staining, the nuclei were stained with hematoxylin in blue and the cytoplasm was stained by eosin in pink. The PBS-treated and both aptamer-treated groups showed rhombic or polygonal cells with large spherical or spindle-shaped nuclei, which indicating the normal cells without apoptosis and necrosis (Fig. 7d ). Fig. 7 The effect of NucA modification on the antitumor activity of the conjugated PTX. a Macroscopic views of the xenografted tumor after 4 weeks of different treatments from the groups indicated. Scale bar, 1 cm. b Analysis of tumor volume after 4 weeks of different treatments indicated at a dosing frequency of twice a week via intravenous injection. The dosing points were indicated with blue arrows. The data were presented as the means ± standard deviation. n = 6, * P < 0.05. c Ki-67 immunohistochemical staining analysis of ovarian tumor sections from the groups indicated. Ki-67-positive staining was indicated by brown and nuclei were stained by blue. Scale bars, 100 μm. d H&E staining analysis of ovarian tumor sections from each group. Arrows indicate cell apoptosis and necrosis in the tumor sections. Scale bars, 100 μm. Note: PBS, the xenografted mice treated with PBS. PTX, the xenografted mice treated with paclitaxel. CRO, the xenografted mice treated with CRO aptamer. NucA, the xenografted mice treated with nucleolin aptamer. CRO-PTX, the xenografted mice treated with CRO-PTX. NucA-PTX, the xenografted mice treated with NucA-PTX Full size image The effect of NucA modification on in vivo toxicity Considering the toxicities of paclitaxel (e.g., hematological toxicity and neurotoxicity) reported in clinical application, we further evaluate the toxicity of NucA-PTX in the xenografted mouse model. First, we measured the body weight of the treated mice every 4 days during the treatments. PTX-treated group showed obvious weight loss (about 85%) throughout the experiment, indicating the potential of systematic toxicity. In contrast, no remarkably body weight loss was observed in PBS-, CRO-, NucA-, and NucA-PTX-treated groups, revealing a slightly low potential of systemic toxicity (Fig. 8a ). Next, we investigated the myelosuppression of NucA-PTX through white blood cell (WBC) count test. No obvious change of WBC count was observed in xenografted mice after treatment with PBS and CRO, whereas PTX and CRO-PTX induced a significant decrease in the value of WBC count. The value of WBC count in the NucA-PTX-treated mice was also decreased compared with the value before administration but to a much lesser extent than that in PTX-treated group (Fig. 8b ). Furthermore, we evaluated the potential neurotoxicity of NucA-PTX using an electromyography apparatus. PTX and CRO-PTX induced a marked and significant reduction in caudal and digital nerve conduction velocities (NCVs) when compared to the PBS- and CRO-treated groups, hinting the potential neurotoxicity of PTX. NucA-PTX also induced caudal and digital NCVs reduction compared to PBS control group, but the value of NCVs was higher than that in CRO-PTX-treated group (Fig. 8c ). Finally, The PTX-related toxicities to major organs were evaluated by histology analysis with H&E staining and serum biochemical assay, respectively. As expected, serious damages were observed in the H&E-stained sections of heart, liver, spleen, and lung, respectively, in the xenografted mice with PTX- and CRO-PTX treatment (Fig. 8d ). For heart damage, myofibrillar loss and atrophy of myocardial cells were found. For liver damage, hepatic cords loss, mild steatosis, and dilatayion of blood sinus were observed. For lung injury, broken lung fibers were found. For spleen damage, the atrophy of the white pulp was detected. However, the above damages to these tissues was greatly reduced or absent in NucA-PTX treated group when compared to those in PTX and CRO-PTX treated groups. Consistently, the histological scores of liver, kidney, lung, heart, and spleen were all significantly lower in the NucA-PTX-treated mice as compared to the mice treated with PTX or CRO-PTX (Fig. 8d ). Interestingly, there is no visible damage in kidneys from all the groups (Fig. 8d, e ). 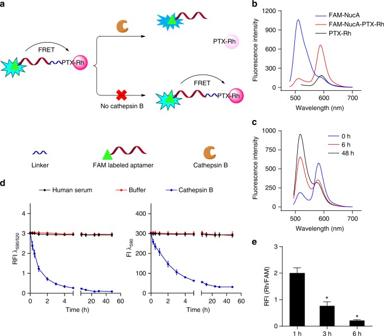Fig. 2 The cathepsin B-dependent release of PTX in FAM-NucA-PTX-Rh.aSchematic diagram of the utilization of FRET in FAM-NucA-PTX-Rh for tracking the rupture of the cathepsin B-labile linker.bFluorescence emission spectra of FAM-NucA-PTX-Rh, FAM-NucA and PTX-Rh (λex = 470 nm). All compounds were at a concentration of 2 μM.cFluorescence emission spectra of FAM-NucA-PTX-Rh (λex = 470 nm) in the presence of cathepsin B upon time. FAM-NucA-PTX-Rh and cathepsin B were at a concentration of 2 μM and 0.5 unit mL−1, respectively.dThe fluorescence analysis of FAM-NucA-PTX-Rh in human serum and buffer (pH 5.0, containing DTT) without or with cathepsin B upon time. The relative fluorescence intensity of rhodamine to FAM (RFIλ590/λ520) indicates the concentration of FAM-NucA-PTX-Rh, and the fluorescence intensity of rhodamine (FIλ590) indicates the concentration of the conjugated PTX-Rh. FAM-NucA-PTX-Rh and cathepsin B were at a concentration of 2 μM and 0.5 unit mL−1, respectively. Error bars indicate mean ± standard deviation.n= 3.eThe intracellular release of PTX-Rh from FAM-NucA-PTX-Rh in SKOV3 cells monitored by flow cytometry. The relative median fluorescence intensity of rhodamine to FAM (RFI Rh/FAM) in SKOV3 cells was examined 1, 3, and 6 h after incubation with 200 nM FAM-NucA-PTX-Rh. Error bars indicate mean ± standard deviation.n= 3, *P< 0.05 Moreover, serum biochemical assays showed that the levels of liver function enzymes, i.e., aspartate aminotransferase (AST) and alanine aminotransferase (ALT), and cardiac function enzymes, i.e., creatine phosphokinase (CPK) and creatine kinase myocardial bound (CK-MB) were all significantly lower in the NucA-PTX-treated mice as compared to the mice treated with PTX or CRO-PTX (Supplementary Table 2 ). Moreover, the serum cytokine levels (TNF-α, INF-γ, IL-1β, IL-6, IL-10) of both nude mice (immune-incompetent) and Balb/c mice (immune-competent) after NucA-PTX treatment was assessed and no notable change in levels was observed in both species (Supplementary Fig. 27 ). Fig. 8 The effect of NucA modification on the toxicity of the conjugated PTX. a Body weight changes after 4 weeks of different treatments indicated in xenografted mice. Body weight was normalized to each body weight before treatment. The dosing points were indicated with blue arrows. b The white blood cell count determined by automated hematology analyzer before and after different treatments in xenografted mice. c Neurophysiological analysis of caudal NCV and digital NCV in the xenografted mice 4 days before the end of the different treatments indicated. d Histological assessments of tissues using H&E staining in different treatment groups. Arrows in Heart images indicate the myofibrillar loss and atrophy of myocardial cells. Arrows in Liver images indicate the hepatic cords loss, steatosis and dilatation of blood sinus. Arrows in Spleen images indicate the white pulp atrophy. Arrows in Lung images indicate the broken lung fibers. Scale bars, 100 μm. e Semi-quantitative histological analysis of the H&E-stained tissue sections in different treatment groups. Note: PBS, the xenografted mice treated with PBS. PTX, the xenografted mice treated with paclitaxel. CRO, the xenografted mice treated with CRO aptamer. NucA, the xenografted mice treated with nucleolin aptamer. CRO-PTX, the xenografted mice treated with CRO-PTX. NucA-PTX, the xenografted mice treated with NucA-PTX. The data were presented as the means ± standard deviation. n = 6, * P < 0.05 vs. NucA-PTX group Full size image To connect PTX with the tumor-targeting NucA, the active 2′- hydroxyl group on PTX was the optimal site for substitution. However, it was reported that the introduction of other functional groups on this site resulted in the loss of antitumor activity for the obtained PTX derivatives [25] . Thus, the cathepsin B-labile dipeptide linker was utilized to facilitate the intracellular release of PTX from the conjugate [21] , [24] . In addition, spacers (PABC on PTX side and succinic acid on NucA side) were incorporated to the linker for reducing the steric hindrance for cathepsin B. Previously reported antibody-drug conjugate with the similar dipeptide linker was shown to release drug efficiently in tumor tissues [27] . By monitoring the FRET change of the dual fluorophore-labeled conjugate FAM-NucA-PTX-Rh, our in vitro results demonstrated that the dipeptide linker exhibited remarkable stability in human serum, and the release of PTX was observed either upon addition of cathepsin B or inside tumor cells (Fig. 2 ). In vivo fluorescence analysis of the fluorophore-labeled conjugates in tumor tissue also suggested that the linker still remained intact when initially reaching the tumor site, and then gradually ruptured and released PTX once inside tumor cells (Supplementary Fig. 26 ). The cellular uptake of NucA-PTX-Rh was shown in a nucleolin-dependent manner and significantly higher in cancer cells, while the uptake of CRO-PTX-Rh was moderate and did not exhibited notable difference in cell lines with various surface nucleolin expression levels, suggesting that the interaction between NucA and nucleolin played a crucial role in the entrance of the conjugated PTX into cancer cells. NucA-PTX-Rh was mainly taken up by cancer cells through macropinocytosis, which is consistent with the findings previously reported that macropinocytosis was the endocytic pathway of AS1411 [28] . In contrast, the endocytosis of CRO-PTX-Rh in cancer cells and NucA-PTX-Rh in normal cells were relatively non-specific and no clear pathways was noted. As macropinosomes would finally fused into lysosomes [29] , the co-localization of NucA-PTX-Rh and lysotracker was also observed in this study. Lysosomes are the intracellular sites where cathepsin B is most abundant and active at its optimal pH (4.5−5.0) [22] . The localization of NucA-PTX-Rh in lysosomes suggests that the intracellular environment would be suitable for the sufficient cleavage of the cathepsin B-labile linker in cancer cells. Compared to its CRO counterpart, NucA-PTX exhibited higher cytotoxicity in cancer cells but lower cytotoxicity in normal cells, which was consistent with the uptake results. It was notable that CRO-PTX showed a certain amount of uptake and a moderate cytotoxicity in cancer cells in vitro, in the meanwhile NucA-PTX had a low level of uptake and a slight cytotoxicity in normal cells at high concentrations in vitro. This could possibly because during the in vitro incubation, there were non-specific interactions between aptamers and cell surfaces regardless of aptamer sequence or nucleolin expression level, and the selectivity of NucA to cancer cells may stand out in vivo when both tumor and normal cells were presented. Accordingly, in the human ovarian cancer xenografted mouse model, the NucA modification facilitated the accumulation of the conjugated PTX in tumor tissue rather than major organs, subsequently resulting in improved antitumor efficacy—smaller tumor size and less active proliferation in tumor tissue than CRO-PTX treated mice. Emerging evidence showed that PTX chemotherapy induces severe hematologic toxicities (neutropenia and leukopenia) and organ damages [30] , [31] . Neurotoxicity of PTX is also a clinical challenge, and cancer patients receiving PTX treatment may develop peripheral neuropathies [32] , [33] . In our studies, no significant WBC toxicity, neurotoxicity and major organ damage were observed in mice treated with NucA-PTX compared to that treated with PTX or CRO-PTX. The improved efficacy and reduced toxicity of NucA-PTX in vivo was most likely attributed to the stability of the linker in circulation and the selective accumulation in tumor tissues with high nucleolin expression led by NucA. AS1411, the same sequence as NucA, has been reported with tumor growth inhibition and utilized in phase II clinical trials [20] . However unexpectedly, no activity was observed for NucA either in vitro or in vivo in our studies. This could be explained by the following possible reasons. For in vitro cytotoxicity study, the concentration range that we examined was set based upon the activity of PTX, which was within nanomolar range [34] . While AS1411 was reported to be cytostasis and only inhibit the growth of cancer cells in micromolar range [35] , [36] . In addition, the induction of cell death by AS1411 occurs only after prolonged exposure to AS1411 and varies from different cell lines [35] . For in vivo anti-cancer efficacy studies, normally a continuous infusion of AS1411 at a relative high dose for 4 or 7 days was chosen as the route of administration for clinical studies [35] . However, the in vivo dose used in our study was also set according to PTX [37] , [38] , [39] , [40] , which was lower and less frequent—twice a week. Besides, ovarian cancer was probably not among the most sensitive cancer types to AS1411 compared to acute myeloid leukemia, or metastatic renal cell carcinoma, which were chosen as indications of AS1411 for phase II studies [20] , [35] . Thus, it is reasonable that we did not observe anti-cancer activities for NucA in our studies. Other investigators have reported utilizing the nucleolin aptamer as a targeting ligand on nanoparticles for PTX delivery [37] , [38] , [39] , [40] . Guo et al. [37] developed AS1411-functionalized PEG-PLGA nanoparticles and enhanced the accumulation of PTX in glioma. AS1411 modified pH-sensitive micelles [38] and AS1411 modified HSA protein nanoparticles [39] were also investigated for tumor targeted delivery of PTX. However the inhomogeneity, instability, immunogenicity, and potential toxicity of those nanoparticles or their lipid/polymer materials remain concerns [41] , [42] . By contrast, our NucA-PTX as a single macromolecule with direct connection of the nucleolin aptamer with paclitaxel, exhibits great improvements in terms of these properties. In addition to excellent stability and homogeneity, our studies also revealed the lack of immunogenicity and toxicity for NucA-PTX, which represents a step further toward the clinical translation for aptamers. As alternatives of ADCs, this work establishes an innovative technology platform for ApDC development. Moreover, by altering aptamers that target different cancer cells (e.g., Her2 positive breast cancer cells, triple negative breast cancer cells, non-small cell lung cancer cells, osteosarcoma cells, and so on), the personalized paclitaxel derivatives could be developed for the patients with the according cancer types. Importantly, it provides an efficient approach to the next-generation of smart antitumor drug discovery toward precision medicine, i.e., personalized aptamer-drug conjugates. Cell culture Human ovarian cancer cell lines SKOV3 (ATCC HTB-77) and OVCAR3 (ATCC HTB-161) were purchased from American Type Culture Collection (ATCC, USA). Human normal liver cell line L02 was purchased from China Center for Type Culture Collection (CCTCC, China). The cells were maintained in ATCC-formulated DMEM (for SKOV3 and OVCAR3) or RPMI-1640 (for L02) medium, supplemented with 10% fetal bovine serum, 1% penicillin-streptomycin, and incubated at 37 °C with 5% CO 2 and 95% humidity. The cell lines were negative for mycoplasma. Paclitaxel intracellular release SKOV3 cells were seeded in a 24-wells plate at a density of 2 × 10 5 cells each well and incubated overnight. FAM-NucA-PTX-Rh at a concentration of 200 nM was added to the media of cells for 1 h incubation. The cells were then washed and re-suspended in culture medium, analyzed immediately, or at 3 h and 6 h by a FACScan cytometer (BD 831 Immunocytometry Systems). Cellular uptake of aptamer-PTX conjugates in vitro SKOV3 cells were seeded in a 24-well plate at a density of 2 × 10 5 cells per well and incubate overnight. For time-dependent uptake experiment, NucA-PTX-Rh or CRO-PTX-Rh were added to a final concentration of 500 nM. After 1, 2, 3, 4, 5, and 6 h of incubation, the cells were washed three times with PBS, trypsinized and re-suspended in 400 μL PBS after centrifugation (1000 r.p.m., 5 min). The fluorescence intensity of rhodamine was determined with a FACScan cytometer (BD 831 Immunocytometry Systems) by counting 10,000 events. SKOV3 cells without any drug incubation were performed as a blank control to measure background signals which were subtracted from the final calculations. For concentration-dependent uptake assay, the final concentration of NucA-PTX-Rh and CRO-PTX-Rh was 60 nM, 120 nM, 250 nM, 500 nM, and 1 μM, respectively. After 2 h of incubation, the same procedures were conducted as the time-dependent uptake experiment. The experiments were performed with triplicates and were repeated for three times. For nucleolin-dependent uptake assay, SKOV3, OVCAR3, and L02 cells were incubated with Alexa 488-labeled-nucleolin antibody, NucA-PTX-Rh or CRO-PTX-Rh for 2 h. The cells were then centrifuged, washed and re-suspended for analysis by flow cytometry. For aptamer blocking experiment, the SKOV3 cells were pre-incubated with 250 nM either NucA or CRO for 2 h, and then incubated with 100 nM NucA-PTX-Rh for 2 h. The cells were then centrifuged, washed and re-suspended for analysis by flow cytometry. Gating strategy of flow cytometry analysis is shown in Supplementary Fig. 21 . Confocal imaging for endocytosis pathways SKOV3 or L02 cells were seeded in glass bottom confocal dishes at a density of 5 × 10 4 per well and incubated overnight. Cells were then incubated with 250 nM of NucA-PTX-Rh or CRO-PTX-Rh and Alexa Fluor 488-labeled endocytic markers (25 μg mL −1 dextran, 25 μg mL −1 transferrin and 5 μg mL −1 CTX-B) at 37 °C for 2 h. Volume of 2 μg mL −1 Hoechst 33,342 then was added during the final 15 min of the incubation. After 2 h of incubation, the cells were washed and visualized by confocal microscopy. To investigate the sub-cellular trafficking, the cells were incubated with 250 nM of NucA-PTX-Rh or CRO-PTX-Rh at 37 °C for 1 h. 75 nM LysoTracker Green DND-26 (Invitrogen) was added to the cells for another 1 h. Volume of 2 μg mL −1 Hoechst 33,342 then was added during the final 15 min of the incubation. After 2 h of incubation, the cells were washed and visualized by confocal microscopy. Chemical inhibition of endocytosis pathways SKOV3 or L02 cells were seeded in 6-well plates at a density of 5 × 10 5 cells per well and incubated overnight. The cells were then pre-incubated with the inhibitor of macropinocytosis (EIPA), the inhibitor of clathrin pathway (Chlorpromazine) or the inhibitor of caveolae pathway (Filipin) at various concentrations for 30 min prior to the addition of NucA-PTX-Rh or CRO-PTX-Rh at a concentration of 500 nM. After 2 h, the cells were trypsinized, centrifuged (1000 r.p.m., 5 min) and the supernatants were removed. After washed twice with PBS, the cells were re-suspended in 400 μL of PBS. Fluorescence was determined with a FACScan cytometer (BD 831 Immunocytometry Systems) by counting 10,000 events. SKOV3 or L02 cells with DMSO were performed as a blank control to measure background signals which were subtracted from the final calculations. In vitro cell viability assay The cell viability assay was conducted using a Cell Counting Kit-8 (CCK8, Dojindo). According to the provided protocol, SKOV3, OVCAR3, and L02 cells were seeded in 96-well plates with ~5000 cells in each well and incubated overnight for adherence. Solutions of 500 nM NucA, CRO, PTX, NucA-PTX, and CRO-PTX were made up in medium and a serial twofold dilution of the solution were performed to achieve a range of concentrations from 15.6 to 500 nM. The media of cells were removed and the solutions were added for 24 h or 72 h incubation at 37 °C. At the end of the incubation, 10 µL of CCK8 solution was added to each well. The plates were read after additional 3 h incubation by a spectrometer at 450 nm. IC 50 values of 72 h were calculated using Graph Pad based on the viability curve data. Cell cycle assay Cell cycle analysis was performed by following the instructions of the Propidium Iodide Flow Cytometry Kit (abcam). Briefly, SKOV3 and OVCAR3 cells (5 × 10 5 per well) were seeded in 6-well plates and incubated overnight. After washing with PBS, the cells were incubated with 200 nM PTX, NucA-PTX or CRO-PTX at 37 °C for 48 h. At the end of incubation, the cells were trypsinized, washed, and fixed in 66% ethanol on ice. After storage at 4 °C overnight, the cells were washed, re-suspended in 200 μL. 1 × Propidium Iodide + RNase Staining Solution and incubated at 37 °C in the dark for 30 min. Finally, DNA content was measured by Flow Cytometry (BD 831 Immunocytometry Systems), the percentage of cells in each phase of the cell cycle was calculated using the ModFit software. 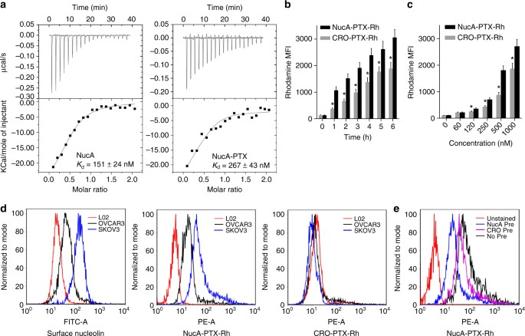Fig. 3 The effect of NucA modification on the uptake of the conjugated PTX-Rh.aThe interaction of nucleolin with NucA and NucA-PTX, respectively, detected by isothermal titration calorimetry (ITC). NucA or NucA-PTX was injected into nucleolin at a 10:1 ratio in 19 portions (each portion 2 μL) at 25 °C.bThe time-dependent cellular uptake of the conjugated PTX-Rh in SKOV3 cells examined by flow cytometry. SKOV3 cells were incubated with either NucA-PTX-Rh or CRO-PTX-Rh at a concentration of 500 nM for 1 to 6 h. Error bars indicate mean ± standard deviation.n= 5, *P< 0.05.cThe concentration-dependent cellular uptake of the conjugated PTX-Rh in SKOV3 cells examined by flow cytometry. SKOV3 cells were incubated with either NucA-PTX-Rh or CRO-PTX-Rh at a range of concentrations for 2 h. Error bars indicate mean ± standard deviation.n= 5, *P< 0.05.dThe nucleolin expression on cell surface, and the uptake of NucA-PTX-Rh or CRO-PTX-Rh in SKOV3, OVCAR3 and L02 evaluated by flow cytometry. The cells were treated with NucA-PTX-Rh or CRO-PTX-Rh at a concentration of 100 nM for 2 h. The nucleolin expression was detected using Alexa488-labeled anti-nucleolin antibody shown in the FITC channel, and the rhodamine level of the conjugates was shown in the PE channel.eThe cellular uptake of NucA-PTX-Rh in SKOV3 pre-incubated with either NucA (NucA Pre) or CRO (CRO Pre) analyzed by flow cytometry. The cells were pretreated with 250 nM NucA or CRO for 2 h before incubated with 100 nM NucA-PTX-Rh for 2 h. The rhodamine level of NucA-PTX-Rh was shown in the PE channel Animal handing The mice were housed in Laboratory Animal House of Hong Kong Baptist University. The animal house is temperature-controlled with a 12 h light/dark cycle. Food and water were available ad libitum. At least a week’s adaptation was given to mice before starting any experiments. The procedures of all in vivo studies have gained ethics approval by the Animal Experimentation Ethics Committee of the Hong Kong Baptist University. Mice modeling Eight-week-old female BALB/c nude mice were inoculated subcutaneously with 2 × 10 6 SKOV3 cells in the left armpit. Tumors were observed 2 weeks after inoculation. The tumor-bearing nude mice were randomly divided into groups with six mice in each group for further studies. Tissue distribution by biophotonic imaging analysis NucA-PTX-Rh and CRO-PTX-Rh at a single dose of 5 mg kg −1 were given to two groups of the tumor-bearing nude mice, respectively, by intravenous route (i.v.) 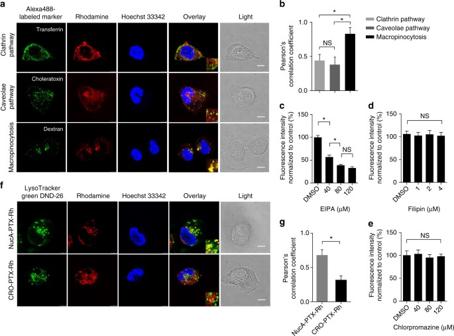Fig. 4 The effect of NucA modification on cellular internalization and trafficking.aRepresentative images showing the co-localization of the conjugated PTX-Rh (red) in NucA-PTX-Rh with Alexa Fluor 488-labled endocytic markers (transferrin, choleratoxin and dextran; green) by confocal microscopy. The nuclei were counterstained with Hoechst 33,342 (blue). Scale bar, 10 μm.bPearson’s correlation coefficient analysis of the co-localization between NucA-PTX-Rh and endocytosis markers in SKOV3 cells by Image J Coloc2. Error bars indicate mean ± standard deviation.n= 5 per group. Each replicate is from one biological experiment, quantified with 10 independent fields of view. *P< 0.05; NS: not significant difference.c-eThe chemical inhibition of cellular uptake for the conjugated PTX-Rh in CRO-PTX-Rh in SKOV3 cells. The relative fluorescence of rhodamine was quantified after the treatment with inhibitors of three endocytic pathways by flow cytometry: EIPA (macropinocytosis,c), Filipin (caveolae pathway,d), and Chlorpromazine (clathrin pathway,e). Error bars indicate mean ± standard deviation.n= 3. *P< 0.05; NS: not significant difference.fRepresentative images showing the co-localization of the conjugated PTX-Rh (red) with a lysosomal marker (LysoTracker Green DND-26; green) by confocal microscopy. The nuclei were counterstained with Hoechst 33,342 (blue). Scale bar, 10 μm.gPearson’s correlation coefficient analysis of the co-localization between the conjugates and lysotracker in SKOV3 cells by Image J Coloc2. The data were presented as the means ± standard deviation.n= 5 per group. Each replicate is from one biological experiment, quantified with 10 independent fields of view. *P< 0.05 via the tail vein. The mice were killed 2 h and 4 h after injection. Tumors and major organs (hearts, lungs, livers, spleens, and kidneys) were collected for biophotonic imaging. Biophotonic imaging was performed using an IVIS Lumina XR imaging system. All images were acquired with an exposure time of 5 s. The distribution of fluorescence within tissues was represented as a pseudo-color image. The photographic and fluorescent images were individually acquired and then overlaid. Ex vivo localization of NucA-PTX-Rh in liver, kidney, and tumor sections The liver, kidney, and tumor tissues were collected and placed in 4% paraformaldehyde leaving for overnight. The tissues were then incubated in 30% sucrose for 6 h, before embedding in optimal cutting temperature medium (OCT). The embedded tissues were then cryosectioned, washed, and permeabilized by 0.1% Triton X-100. Finally, the sections were stained with Alexa Fluor 488 Phalloidin (Invitrogen) and mounted with ProLong Antifade Reagent with DAPI (Molecular Probes). A total of six sections of the liver and kidney from each mouse were randomly selected for immunostaining and image acquisition by a confocal microscopy, respectively. To determine the co-localization of PTX-Rh with nucleolin-expressing tumor cells, the Pearson’s coefficient analysis were performed on the fluorescent micrographs of tumor cryosection by ImageJ software (National Institutes of Health, USA). To determine the distribution of PTX-Rh in liver and kidney, the percentage of rhodamine positive nephrocytes and hepatocytes per microscopic view were calculated from the confocal images of six different views per section with the ×20 microscope objective. Percentage of injected doses NucA-PTX-Rh and CRO-PTX-Rh at a single dose of 5 mg kg −1 were given to two groups of the tumor-bearing nude mice, respectively, by intravenous route (i.v.) via the tail vein. The mice were killed 2 h and 4 h after injection. 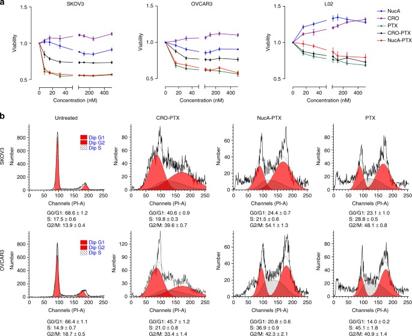Fig. 5 The effect of NucA modification on the cytotoxicity of the conjugated PTX.aThe cell viabilities of SKOV3, OVCAR3, and L02 after 24 h treatment of NucA, CRO, PTX, CRO-PTX, or NucA-PTX evaluated by CCK8 assay. The concentration range of each compound was from 15.6 to 500 nM. The data were presented as the means ± standard deviation.n= 3.bThe cell cycle distribution of SKOV3 and OVCAR3 cells after 48 h treatment of CRO-PTX, NucA-PTX, or PTX analyzed by flow cytometry Tumors and major organs (hearts, lungs, livers, spleens, and kidneys) were collected, weighed, chopped, and homogenized. The rhodamine fluorescence of the tissue homogenates were analyzed by a fluorescence spectrophotometer. Tumor and organ homogenates from untreated mice were used as blank controls. The fluorescence intensity of NucA-PTX-Rh and CRO-PTX-Rh at injected dose was measured as the 100% standard. Percentage of injected doses of tumor and each organ were calculated based upon the relative fluorescence intensities. Intactness of the conjugate at tumor site in vivo NucA-PTX-Rh and FAM-NucA-PTX-Rh at a single dose of 5 mg kg −1 were given to the tumor-bearing nude mice, respectively, by intravenous route (i.v.) via the tail vein. The mice were killed at 0.5, 1, 1.5, 2, 2.5, 3, 3.5, and 4 h. The tumors were then collected, chopped and homogenized. The fluorescence of rhoamine in NucA-PTX-Rh treated mouse tumor homogenates and the fluorescence of rhodamine and FAM in FAM-NucA-PTX-Rh treated mouse tumor homogenates were analyzed by a fluorescence plate reader. Plasma half-life NucA-PTX-Rh at a single dose of 5 mg kg −1 was given to the tumor-bearing nude mice by intravenous route (i.v.) via the tail vein. The rhodamine fluorescence in plasma at various time points were measured. The fluorescence at 0 h was estimated by adding given dose of NucA-PTX-Rh to full volume plasma from a mouse. The plasma clearance curve was presented by the relative fluorescence intensities of the conjugate over time and the plasma half-life ( t 1/2 ) was calculated by performing a logarithm plot. In vivo antitumor efficacy evaluation CRO, NucA, NucA-PTX, CRO-PTX, or PTX at a dosage of 2.4 μmol kg −1 (with the equivalent PTX concentration of 2 mg kg −1 ) were given to mice of five groups by i.v. twice a week for 4 weeks. Another group were given vehicle solution PBS as the control group. The tumor size and body weight were monitored every 4 days. At the end of the treatment, the mice were killed, blood was collected for WBC count analysis and biochemical analysis. The tumors and major organs (hearts, lungs, livers, kidneys, and spleens) were collected for immunohistochemistry and/or histological examinations. Immunohistochemistry Paraffin sections of tumors were deparaffinized using xylene, and then rehydrated by immersing in alcohol at series of concentrations. Endogenous peroxidase was quenched by 10 min incubation with 3% hydrogen peroxide. Blocking serum of 1:10 was used for blocking the non-specific bindings of epitopes. The sections were incubated with mouse Ki-67 antibody (Abcam) of 1:100 at 4 °C overnight. The slides were washed three times, incubated with a biotinylated secondary antibody (sc-7207; Santa Cruz Biotechnology) for 30 min and then with peroxidase substrate for 10 min. The sections were finally washed, incubated in deionized water for 5 min, counter stained with hematoxylin before analyzing by microscopy (Leica DMRB DAS; Leica, Switzerland). Histological examination Isolated tissues and organs including the xenografted tumors, hearts, lungs, livers, kidneys, and spleens were fixed in 10% neutral-buffered formalin followed by embedding in paraffin. Five micrometer section was made, mounted on glass slides, deparaffinized, and subjected to hematoxylin and eosin (H&E) staining using standard protocols. After mounting with coverslips, the specimens were viewed and blindly analyzed by a pathologist under a light microscope (Leica DMRB DAS; Leica, Heerbrugg, Switzerland). The qualitative analysis was performed as previously reported [43] , [44] , [45] . Moreover, the histological grading systems were applied for the semi-quantitative analysis of the damages in the sections of liver, kidney, lung, heart, and spleen, respectively. Briefly, the liver sections were scored ranging from 0 to 2, or 3 depending on the changes in hepatocytes and hepatocyte rows as well as the presence of steatosis, fibrosis, necrosis, macrophages, and lymphocytes [46] . The kidney sections were scored ranging from 0 to 2, or 3 depending on the changes in glomeruli, tubular structure, epithelial cells, and medulla, as well as the presence of fibrin deposition, vascular dilation, inflammatory cells, fibrosis, and necrosis [46] . The lung sections were graded by a 4-point scoring method regarding the inflammatory changes of the lung tissue, hemorrhage in the alveolar cavity, and edema and thickening of the alveolar wall [47] . The heart sections were graded with a maximum score of 5 according to the morphological changes in myocardial cell [48] . The spleen sections were graded with a maximum score of 12 according to inflammation, necrosis/abscess formation and thrombus formation [49] . Neurophysiological assessment The effect of treatments on neurophysiology of mice were assessed by determining the caudal and digital nerve conduction velocities (NCVs) as previously reported [50] . Briefly, for monitoring caudal NCV, the recording needle electrodes were placed at the base of the tail and the stimulating needle electrodes were positioned 3.5 cm distally. For monitoring digital NCV, the recording electrodes were placed near the ankle and the stimulating electrodes were positioned closed to the fourth toe on the same leg. The distances between stimulating and recording electrodes were measured. The latency of responses was recorded using an electromyographic instrument (Myto2 ABN Neuro, Italy). For each recording ten responses were averaged. The NCVs were calculated based on the formula: the distance/the latency. Immune response assessment Immune response of NucA-PTX in Balb/c nude mice or Balb/c mice was examined after 4-week treatment of NucA-PTX (intravenous administration twice a week). A control group was set by given PBS instead of NucA-PTX. At the end of the treatment, the mice were killed and sera were collected. Levels of serum TNF-α, IFN-γ, IL-1β, IL-6, and IL-10 were determined by ELISA Kits (Abcam) and normalized to the PBS control group. Biochemical assays for liver and cardiac function enzymes The levels of two liver function enzymes: aspartate aminotransferase (AST) and alanine aminotransferase (ALT) were analyzed by ELSA kits (Abcam for AST and Cusabio Biotech for ALT). For two cardiac function enzymes, creatine phosphokinase (CPK) was analyzed by Creatine Kinase Activity Assay Kit (Abcam), and creatine kinase myocardial bound (CK-MB) was analyzed by Mouse Creatine Kinase MB isoenzyme (CK-MB) ELISA Kit (Cusabio Biotech). 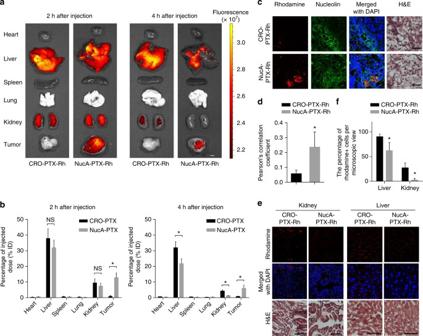Fig. 6 The effect of NucA modification on the distribution of the conjugated PTX-Rh.aThe distribution of the conjugated PTX-Rh in tumor and major viscera (heart, liver, spleen, lung, and kidney) at organ level 2 h and 4 h after intravenous injection of NucA-PTX-Rh or CRO-PTX-Rh visualized by biophotonic imaging.bPercentage of injected dose in tumor and major viscera 2 h and 4 h after intravenous injection of NucA-PTX-Rh or CRO-PTX-Rh evaluated by measuring the fluorescent intensity of rhodamine. The data were presented as the means ± standard deviation.n= 6, NS: not significant, *P< 0.05.cThe representative fluorescent micrographs of the distribution of the conjugated PTX-Rh in tumor at tissue level 4 h after intravenous injection of NucA-PTX-Rh or CRO-PTX-Rh examined by confocal microscopy. NucA-PTX-Rh and CRO-PTX-Rh were indicated by rhodamine (red). Immunofluorescence staining was performed by Alexa488-labeled anti-nucleolin antibody (green). Merged images with DAPI staining show co-localization of the conjugates with nucleolin positive cells. H&E staining images were from the same cryosections. Scale bars, 80 μm.dThe Pearson’s coefficient analysis for the distribution of the conjugated PTX-Rh (red) with nucleolin-expressing tumor cells (green).eRepresentative fluorescent micrographs of the distribution of the conjugated PTX-Rh in kidney and liver at tissue level 4 h after intravenous injection of NucA-PTX-Rh or CRO-PTX-Rh examined by confocal microscopy. NucA-PTX-Rh and CRO-PTX-Rh were indicated by rhodamine (red). Merged images with DAPI staining show rhodamine positive cells. H&E staining images were from the same cryosections. Scale bars, 80 μm.fThe percentage of rhodamine positive cells per microscopic view. Note: CRO-PTX-Rh, the xenografted mice treated with CRO-PTX-Rh. NucA-PTX-Rh, the xenografted mice treated with NucA-PTX-Rh. The data were presented as the means ± standard deviation.n= 4, *P< 0.05 vs. CRO-PTX-Rh group Statistical analysis All the variables were expressed as mean ± standard deviation. 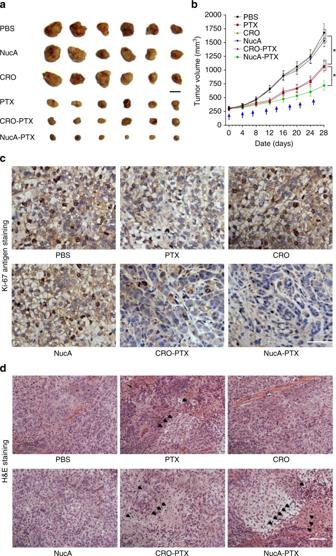Fig. 7 The effect of NucA modification on the antitumor activity of the conjugated PTX.aMacroscopic views of the xenografted tumor after 4 weeks of different treatments from the groups indicated. Scale bar, 1 cm.bAnalysis of tumor volume after 4 weeks of different treatments indicated at a dosing frequency of twice a week via intravenous injection. The dosing points were indicated with blue arrows. The data were presented as the means ± standard deviation.n= 6, *P< 0.05.cKi-67 immunohistochemical staining analysis of ovarian tumor sections from the groups indicated. Ki-67-positive staining was indicated by brown and nuclei were stained by blue. Scale bars, 100 μm.dH&E staining analysis of ovarian tumor sections from each group. Arrows indicate cell apoptosis and necrosis in the tumor sections. Scale bars, 100 μm. Note: PBS, the xenografted mice treated with PBS. PTX, the xenografted mice treated with paclitaxel. CRO, the xenografted mice treated with CRO aptamer. NucA, the xenografted mice treated with nucleolin aptamer. CRO-PTX, the xenografted mice treated with CRO-PTX. NucA-PTX, the xenografted mice treated with NucA-PTX 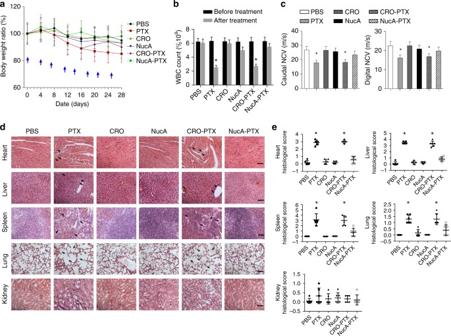Fig. 8 The effect of NucA modification on the toxicity of the conjugated PTX.aBody weight changes after 4 weeks of different treatments indicated in xenografted mice. Body weight was normalized to each body weight before treatment. The dosing points were indicated with blue arrows.bThe white blood cell count determined by automated hematology analyzer before and after different treatments in xenografted mice.cNeurophysiological analysis of caudal NCV and digital NCV in the xenografted mice 4 days before the end of the different treatments indicated.dHistological assessments of tissues using H&E staining in different treatment groups. Arrows in Heart images indicate the myofibrillar loss and atrophy of myocardial cells. Arrows in Liver images indicate the hepatic cords loss, steatosis and dilatation of blood sinus. Arrows in Spleen images indicate the white pulp atrophy. Arrows in Lung images indicate the broken lung fibers. Scale bars, 100 μm.eSemi-quantitative histological analysis of the H&E-stained tissue sections in different treatment groups. Note: PBS, the xenografted mice treated with PBS. PTX, the xenografted mice treated with paclitaxel. CRO, the xenografted mice treated with CRO aptamer. NucA, the xenografted mice treated with nucleolin aptamer. CRO-PTX, the xenografted mice treated with CRO-PTX. NucA-PTX, the xenografted mice treated with NucA-PTX. The data were presented as the means ± standard deviation.n= 6, *P< 0.05 vs. NucA-PTX group Student’s t -test or one-way analyses of variance (ANOVA) were performed in statistical evaluation. A p -value <0.05 was considered to be significant. Data availability All data are available within the Article and Supplementary Files, or available from the authors upon reasonable request.